Metastasis is regulated via microRNA-200/ZEB1 axis control of tumour cell PD-L1 expression and intratumoral immunosuppression Immunosuppression of tumour-infiltrating lymphocytes (TIL) is a common feature of advanced cancer, but its biological basis has remained obscure. We demonstrate here a molecular link between epithelial-to-mesenchymal transition (EMT) and CD8 + TIL immunosuppression, two key drivers of cancer progression. We show that microRNA-200 (miR-200), a cell-autonomous suppressor of EMT and metastasis, targets PD-L1. Moreover, ZEB1, an EMT activator and transcriptional repressor of miR-200, relieves miR-200 repression of PD-L1 on tumour cells, leading to CD8 + T-cell immunosuppression and metastasis. These findings are supported by robust correlations between the EMT score, miR-200 levels and PD-L1 expression in multiple human lung cancer datasets. In addition to revealing a link between EMT and T-cell dysfunction, these findings also show that ZEB1 promotes metastasis through a heretofore unappreciated cell non-autonomous mechanism, and suggest that subgroups of patients in whom malignant progression is driven by EMT activators may respond to treatment with PD-L1 antagonists. Lung cancer is a leading cause of cancer-related mortality, and metastasis is the primary cause of death [1] . Thus, successful prevention of lung cancer mortality requires a thorough understanding of the biological process of metastasis. K-ras LA1/+ p53 R172HΔg/+ ( KP ) mice develop lung cancer that faithfully recapitulates the clinical features of human disease and have been widely used to study lung cancer initiation and progression. We previously showed in this model that microRNA-200 (miR-200) expression is repressed in highly metastatic cancer cells and that forced miR-200 expression reversed the epithelial–mesenchymal transition (EMT) phenotype, abrogating tumour invasion and metastasis [2] , [3] . The significance of these findings is supported by the evidence that low miR-200 expression is part of a microRNA expression signature in primary tumours that predicts disease recurrence in patients with early-stage lung cancer [4] . The miR-200 family includes five members arranged in two genomic clusters (miR-200a/200b/429 and 200c/141) that directly target EMT-inducing transcription factors, including zinc-finger E-box-binding homeobox 1 (ZEB1) (ref. 5 ). In turn, ZEB1 can directly repress the transcription of both miR-200 loci. In cancer cells, the miR-200/ZEB1 axis controls the expression of multiple genes involved in migration, invasion and metastatic growth at distant sites. Thus, miR-200 and ZEB1 form a double-negative feedback loop and function as a key regulatory axis of the EMT programme [6] , [7] , [8] , [9] , [10] . The infiltration of lymphocytes into tumour tissues was initially believed to solely reflect attempts by the immune system to reject cancer cells. However, increasing evidence indicates that immune responses can exert either anti or protumorigenic effects [11] , [12] . Immune cells within the tumour microenvironment, such as tumour-associated macrophages, myeloid-derived suppressor cells and regulatory T cells, may contribute to the formation of a suppressive milieu that protects cancer cells from immune destruction [13] , [14] . Furthermore, although cytotoxic CD8 + tumour-infiltrating lymphocytes (CD8 + TILs) can effectively kill cancer cells [15] , prolonged exposure of CD8 + TILs to cancer cells in the tumour bed can lead to complete or partial loss of their effector function, producing a state commonly referred to as exhaustion [16] . How the tumour microenvironment controls CD8 + TIL function is poorly understood. A growing number of studies indicate that co-inhibitory receptor signalling may play a key role in driving CD8 + T-cell exhaustion [16] , [17] , [18] . Indeed, blocking the interaction between the co-inhibitory receptor PD1 and its ligand PD-L1 (also known as B7-H1, CD274) with antibodies has profound therapeutic effects in some patients with advanced non-small cell lung cancer (NSCLC), renal cancer and melanoma [19] , [20] , [21] . Furthermore, the clinical responses to anti-PD1 antibody therapy appear to correlate with higher PD-L1 expression on cancer cells [21] . Nevertheless, PD-L1 is also expressed on various other cell types in the tumour stroma, can be induced by various factors [22] , [23] and its high expression has been associated with poor survival [17] , [24] , [25] . However, the interplay of tumour-intrinsic and -extrinsic mechanisms controlling PD-L1 expression and consequent CD8 + T-cell dysfunction remains poorly defined. In this study, we investigate the regulation of tumour cell PD-L1 expression by the miR-200/ZEB1 axis, and the subsequent suppression of CD8 + T cells in the tumour microenvironment. We uncover a novel mechanism of tumour-intrinsic regulation of PD-L1 via the miR-200/ZEB1 axis, thus linking an EMT regulatory programme to CD8 + TIL exhaustion and further find that immunosuppression is critical to tumour metastasis. Tumour-intrinsic PD-L1 correlates with miR-200 and EMT We recently described a 76-gene EMT signature from mRNA expression in NSCLC, which is predictive for response of cell lines and patient tumours to targeted and chemotherapeutic agents [26] . Application of this signature to score the EMT status of samples in The Cancer Genome Atlas (TCGA) lung adenocarcinoma dataset [27] ( n =230) revealed robust separation of samples along an EMT spectrum, with significant anticorrelation to the expression of the five miR-200 family members, the mRNA levels of ZEB1/2 and the EMT markers E-cadherin, N-cadherin, vimentin and β-catenin, along with the protein levels of multiple EMT markers (E-cadherin, claudin-7, α-catenin, β-catenin, fibronectin; Fig. 1a ). The expression of PD-L1 was strongly upregulated in tumours with a high mesenchymal score (high EMT score; Fig. 1b ; Spearman ρ =0.527, P <2E−16). Analysis of all the microRNAs that correlate with PD-L1 expression in the TCGA dataset ranked the miR-200 family as the top microRNAs with statistically significant negative correlation, for example, for miR-200b, Spearman ρ =−0.454, P =1.55E−13 ( Fig. 1c , Supplementary Fig. 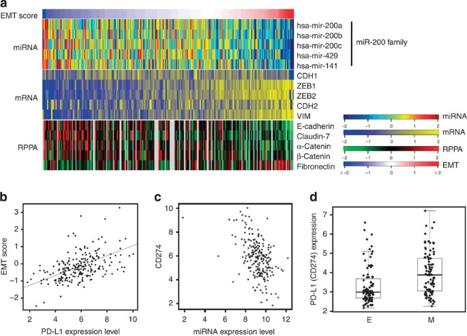Figure 1: EMT correlates with miR-200 and PD-L1 expression in clinical lung cancer datasets. (a) Application of the EMT score (red (right) represents mesenchymal and blue (left) is epithelial) to the lung adenocarcinoma samples from the TCGA dataset (n=230) stratifies the samples by miR-200 family levels (top), EMT marker expression by RNA sequencing (middle), and protein markers (bottom). (b) Dot plot of the concordant EMT score and PD-L1 mRNA expression levels from the samples in the LUAD TCGA. The Spearman correlation is 0.527,P<0.0001. (c) Dot plot of the concordant PD-L1 (CD274) and miR-200b expression levels from the TCGA samples. The Spearman correlation is −0.454,P<0.0001. (d) Application of the EMT score to the samples from the PROSPECT dataset. Samples in the top 1/3 were designated mesenchymal (M) and in the bottom 1/3 designated as epithelial (E). Each group hasn=92 and is represented in the box plot format. The PD-L1 mRNA expression level is graphed for the samples in each group.t-test,P<0.0001. 1 , and Supplementary Table 1 ). Application of the EMT signature to a separate validation set of surgically resected specimens showed statistically higher PD-L1 expression in the samples categorized as mesenchymal ( n =92) versus epithelial ( n =92; P =3.11E−5; Fig. 1d ). These findings suggest that a significant number of primary human NSCLCs express PD-L1 and that the expression correlates with the mesenchymal phenotype of the tumour, as determined by the miR-200 levels. Figure 1: EMT correlates with miR-200 and PD-L1 expression in clinical lung cancer datasets. ( a ) Application of the EMT score (red (right) represents mesenchymal and blue (left) is epithelial) to the lung adenocarcinoma samples from the TCGA dataset ( n =230) stratifies the samples by miR-200 family levels (top), EMT marker expression by RNA sequencing (middle), and protein markers (bottom). ( b ) Dot plot of the concordant EMT score and PD-L1 mRNA expression levels from the samples in the LUAD TCGA. The Spearman correlation is 0.527, P <0.0001. ( c ) Dot plot of the concordant PD-L1 (CD274) and miR-200b expression levels from the TCGA samples. The Spearman correlation is −0.454, P <0.0001. ( d ) Application of the EMT score to the samples from the PROSPECT dataset. Samples in the top 1/3 were designated mesenchymal (M) and in the bottom 1/3 designated as epithelial (E). Each group has n =92 and is represented in the box plot format. The PD-L1 mRNA expression level is graphed for the samples in each group. t -test, P <0.0001. Full size image Tumour cell PD-L1 is regulated by miR-200/ZEB1 axis in NSCLC When transplanted into immunocompetent syngeneic mice, lung adenocarcinoma cell lines derived from K-ras LA1/+ p53 R172HΔG/+ mice ( KP cell lines) produce either highly metastatic, mesenchymal tumours (344SQ and 531LN3) or poorly metastatic, epithelial tumours (393P), properties that are manipulable by ectopic expression of ZEB1 or miR-200b/a/429 (refs 2 , 28 ). To further test the association of PD-L1 with EMT status and the miR-200/ZEB1 axis, we first evaluated the concordant reciprocal changes between PD-L1 and miR-200/ZEB1 expression in vitro . Stable constitutive, inducible or transient miR-200 expression (or conversely, ZEB1 knockdown) suppressed PD-L1 expression on murine (344SQ, 531LN2, 531LN3 and 393P_ZEB1) and human (H157, H1155, H1299 and H460) mesenchymal lung cancer cell lines, while PD-L1 expression was upregulated in non-metastatic epithelial cells (murine 393P and human HCC827) on constitutive ZEB1 expression ( Fig. 2a and Supplementary Figs 2 and 3a,b ). Transforming growth factor-β is a potent EMT inducer that can disrupt the normal ZEB1-miR-200 double-negative feedback loop to drive a mesenchymal phenotype. In both human and murine lung cancer cells treated with transforming growth factor-β, the levels of ZEB1 and PD-L1 were significantly upregulated ( Supplementary Fig. 3c ). 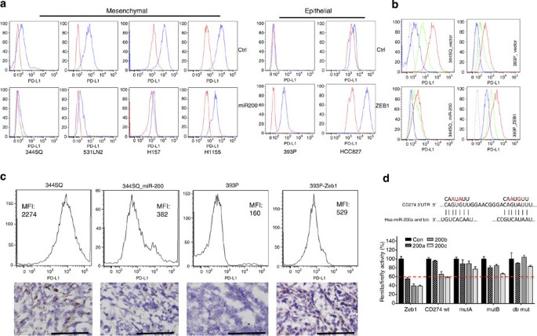Figure 2: PD-L1 levels on human and murine NSCLC cell lines are regulated by the miR-200/ZEB1 axis. (a) Representative fluorescence-activated cell sorting (FACS) histogram of PD-L1 expression on murine (344SQ, 531LN2 and 393P) and human (H157, H1155 and HCC827) lung cancer cells by the overexpression of miR-200 and Zeb1. The analysis was independently repeated three times. (b) The representative FACS histogram of PD-L1 expression on murine lung cancer cells co-cultured with 129/Sv murine splenocytes with or without IFN-γ-neutralizing antibody. Long dash is isotype control staining; blue line is anti-PD-L1 staining without splenocytes; green line is anti-PD-L1 staining with splenocytes blocked by the neutralizing antibody to IFN-γ (20 μg ml−1, 48 h); red line is anti-PD-L1 staining with splenocytes (48 h). The assay was independently performed three times. (c) The representative FACS histogram of PD-L1 (MFI, mean fluorescence intensity) expression in primary subcutaneous tumours grown in syngeneic 129/Sv mice (n=3) injected with the indicated cell lines shown in the upper panel. The representative PD-L1 immunohistochemical staining of each tumour type shown in the bottom panel. Samples were obtained 2 weeks post cell injection. Scale bar, 100 μm. (d) 3′-UTR luciferase reporter assay for WT PD-L1, single (mutant A or B) and double mutants (A and B) versus a Zeb1 3′-UTR control in murine 344SQ cells. The reporters were transiently cotransfected with synthetic miR-200 precursors (200a, 200b or 200c) or control oligomers (con) into 344SQ cells. Values (P<0.05) were normalized based on renilla luciferase and expressed as the mean values (±s.d.) of triplicate wells relative to that of controls cotransfected with empty reporter and empty expression vector or scrambled precursors, which were set at 1.0. The target sequences are shown in the top panel, with the introduced mutations highlighted in red. Figure 2: PD-L1 levels on human and murine NSCLC cell lines are regulated by the miR-200/ZEB1 axis. ( a ) Representative fluorescence-activated cell sorting (FACS) histogram of PD-L1 expression on murine (344SQ, 531LN2 and 393P) and human (H157, H1155 and HCC827) lung cancer cells by the overexpression of miR-200 and Zeb1. The analysis was independently repeated three times. ( b ) The representative FACS histogram of PD-L1 expression on murine lung cancer cells co-cultured with 129/Sv murine splenocytes with or without IFN-γ-neutralizing antibody. Long dash is isotype control staining; blue line is anti-PD-L1 staining without splenocytes; green line is anti-PD-L1 staining with splenocytes blocked by the neutralizing antibody to IFN-γ (20 μg ml −1 , 48 h); red line is anti-PD-L1 staining with splenocytes (48 h). The assay was independently performed three times. ( c ) The representative FACS histogram of PD-L1 (MFI, mean fluorescence intensity) expression in primary subcutaneous tumours grown in syngeneic 129/Sv mice ( n =3) injected with the indicated cell lines shown in the upper panel. The representative PD-L1 immunohistochemical staining of each tumour type shown in the bottom panel. Samples were obtained 2 weeks post cell injection. Scale bar, 100 μm. ( d ) 3′-UTR luciferase reporter assay for WT PD-L1, single (mutant A or B) and double mutants (A and B) versus a Zeb1 3′-UTR control in murine 344SQ cells. The reporters were transiently cotransfected with synthetic miR-200 precursors (200a, 200b or 200c) or control oligomers (con) into 344SQ cells. Values ( P <0.05) were normalized based on renilla luciferase and expressed as the mean values (±s.d.) of triplicate wells relative to that of controls cotransfected with empty reporter and empty expression vector or scrambled precursors, which were set at 1.0. The target sequences are shown in the top panel, with the introduced mutations highlighted in red. Full size image Interferon γ (IFN-γ) is a pleiotropic cytokine that plays a central role in promoting innate and adaptive mechanisms of host defense against a variety of tumours and infectious agents [29] , [30] . Previous reports have established that PD-L1 is upregulated in response to IFN-γ produced by natural killer cells, T cells and macrophages; hence the infiltration of these cells is thought to drive tumour, stromal and myeloid cells to upregulate PD-L1, protecting the tumour from immune attack [25] , [31] . We found that on in vitro IFN-γ stimulation in a co-culture system, the tumour cell expression of PD-L1 was upregulated. Strikingly, the mesenchymal tumour cells (344SQ and 393P_ZEB1) were more responsive to IFN-γ than epithelial tumour cells (344SQ_miR-200 and 393P; Fig. 2b ). The consistent changes in PD-L1 expression on miR-200 or ZEB1 expression observed in vitro were also found in syngeneic KP tumours grown in vivo ( Fig. 2c ). These findings clearly demonstrate that the miR-200/ZEB1 axis plays a dominant role in regulating the tumour cell expression of PD-L1 in either the presence or absence of IFN-γ. The 3′-UTR of PD-L1 contains two very closely approximated sites that are predicted to bind the miR-200 family seed sequences (miR-200a and miR-200b/c; Fig. 2d , Supplementary Fig. 4a and Supplementary Table 2 ), leading us to postulate that PD-L1 is a miR-200 target. Transfection of a wild-type (WT) PD-L1 3′-UTR luciferase reporter construct into murine (344SQ) or human (H157 or H1299) lung cancer cells with low endogenous miR-200 levels revealed luciferase reporter activity that was suppressed on co-transfection of miR-200b or -200c pre-miRs ( Fig. 2d and Supplementary Fig. 4b ), demonstrating a direct regulation of PD-L1 by the miR-200 family members. Mutation of each of the sites partially abrogated the pre-miR recognition, while the double mutant returned the reporter activity to control levels ( Fig. 2d and Supplementary Fig. 4c ). Metastatic phenotype is dependent on CD8 + T-cell function Initially, we found that lung tissues from the genetically engineered K - ras LA1 mice, which develop non-metastatic lung adenocarcinomas, had significantly more CD8 + T cells than lung tissues from the Kras/p53 ( KP ) mice ( Fig. 3a ), in which miR-200 loss drives EMT and metastasis [2] , [3] , [32] . Following subcutaneous or orthotopic intrapulmonary injection into syngeneic, immunocompetent mice, KP cell lines (393P, 344SQ, 393LN, 531LN2) formed tumours with CD8 + T-cell abundances that inversely associated with their metastatic potential ( Fig. 3b and Supplementary Fig. 5a–d ). To examine whether intratumoral CD8 + T-cell suppression promotes tumour growth and metastasis, mice bearing high miR-200 tumours (393P) were treated with control IgG or anti-CD8 antibody to immunodeplete CD8 + T cells, which enhanced tumour growth and metastatic capacity ( Fig. 3c and Table 1 ). As a second approach, 393P or 344SQ cells were injected into syngeneic WT or lymphocyte-deficient Rag 2 −/− mice; metastases were significantly more abundant in Rag2 −/− mice than they were in WT mice ( Fig. 3d and Table 1 ), and adoptive transfer of CD8 + T cells into Rag 2 −/− mice reduced primary tumour growth and suppressed metastasis ( Fig. 3e and Table 1 ). Interestingly, the epithelial and mesenchymal cell types retained their differential metastatic abilities in the Rag2 −/− animals, suggesting an additional role for other cell types, such as natural killer cells. Although it warrants additional investigation, we did not explore this observation further in the current work. 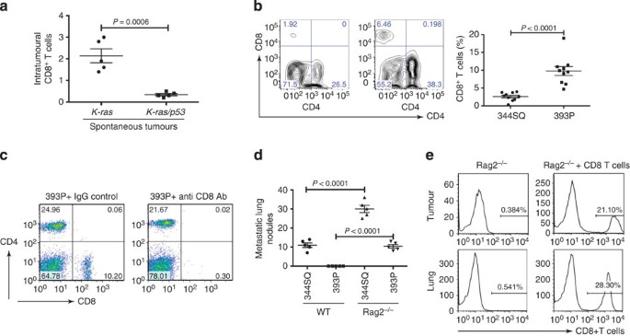Figure 3: CD8+TILs determine the metastatic potential in lung adenocarcinoma models. (a) CD8+T cells measured by flow cytometric analysis in single-cell suspensions prepared from tumour-bearing lungs of 8- to 12- month-oldK-rasLA1/+(K-ras) andK-rasLA1/+p53R172HΔG/+(KP) spontaneous mouse model (n=5). The analysis was independently repeated at least three times.t-test,P=0.0006. (b) The results of a fluorescence-activated cell sorting (FACS) analysis of CD8+TILs in 344SQ and 393P primary tumours isolated 2 weeks after subcutaneous tumour cell injection into 129/Sv mice (n=10). The results contain the data from two independent experiments.t-test,P<0.0001. (c) Representative flow cytometric plot of CD8+TIL numbers from 393P tumour-bearing 129/Sv mice (n=5) treated with anti-CD8 or IgG control antibodies (200 μg, intraperitoneally; twice weekly for 2 weeks beginning on day 1 after a subcutaneous cancer cell injection). (d) Lung metastases in WT or 129/SvRag2−/−mice (n=5) injected subcutaneously with 344SQ or 393P cells and necropsied 5 weeks later. The analysis was independently repeated twice.t-test,P<0.0001. (e) CD8+T cells isolated from 129/Sv mice were adoptively transferred to syngeneic 129/SvRag2−/−mice (n=5). Representative FACS histograms depict the levels of CD8+T cells in 344SQ tumours and lungs of the reconstituted mice with reconstituted CD8+T cells versus those in the controls. Figure 3: CD8 + TILs determine the metastatic potential in lung adenocarcinoma models. ( a ) CD8 + T cells measured by flow cytometric analysis in single-cell suspensions prepared from tumour-bearing lungs of 8- to 12- month-old K-ras LA1/+ ( K-ras ) and K-ras LA1/+ p53 R172HΔG/+ ( KP ) spontaneous mouse model ( n =5). The analysis was independently repeated at least three times. t -test, P =0.0006. ( b ) The results of a fluorescence-activated cell sorting (FACS) analysis of CD8 + TILs in 344SQ and 393P primary tumours isolated 2 weeks after subcutaneous tumour cell injection into 129/Sv mice ( n =10). The results contain the data from two independent experiments. t -test, P <0.0001. ( c ) Representative flow cytometric plot of CD8 + TIL numbers from 393P tumour-bearing 129/Sv mice ( n =5) treated with anti-CD8 or IgG control antibodies (200 μg, intraperitoneally; twice weekly for 2 weeks beginning on day 1 after a subcutaneous cancer cell injection). ( d ) Lung metastases in WT or 129/Sv Rag2 −/− mice ( n =5) injected subcutaneously with 344SQ or 393P cells and necropsied 5 weeks later. The analysis was independently repeated twice. t -test, P <0.0001. ( e ) CD8 + T cells isolated from 129/Sv mice were adoptively transferred to syngeneic 129/Sv Rag2 −/− mice ( n =5). Representative FACS histograms depict the levels of CD8 + T cells in 344SQ tumours and lungs of the reconstituted mice with reconstituted CD8 + T cells versus those in the controls. Full size image Table 1 Primary subcutaneous tumour mass and lung metastases. Full size table miR-200/ZEB1 in tumour cells regulates CD8 + TIL phenotype Tumours of 393P cells expressing ZEB1 demonstrated significantly reduced total CD8 + TILs, an increased percentage of exhausted CD8 + T cells (PD1 + TIM3 + ) ( Fig. 4a,b ), and both increased overall tumour burden (391±24 mg versus 1,194±161 mg) and metastatic lung nodules (0 versus 2.4±0.5). Conversely, ectopic miR-200b/a/429 expression in highly metastatic KP cells (344SQ or 531LN2) increased the numbers of proliferating and granzyme B + CD8 + T cells, decreased the exhausted CD8 + T cells (PD1 + TIM3 + ) and subsequently suppressed metastases ( Fig. 4a–d and Supplementary Fig. 5e ). These effects of ectopic miR-200b/a/429 were reversed by treatment with anti-CD8 antibody ( Fig. 4e,f ) or growth in Rag2 −/− mice ( Fig. 4g ). 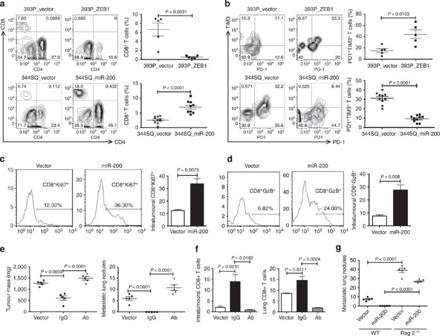Figure 4: The miR-200/ZEB1 axis controls tumour metastasis through regulating CD8+TILs. (a,b) Fluorescence-activated cell sorting analysis of (a) CD8+TIL frequency, (b) PD1 and TIM3 marker expression on CD8+T cells from 393P_vector and 393P_ZEB1 (n=5), as well as 344SQ_vector and 344SQ_miR-200 (n=10) primary tumours. Analysis was done 2 weeks post cancer cell injection. (c,d) Intratumoral Ki67+CD8+T cells (c); granzyme B (GzB)+CD8+T cells (d) in 344SQ_vector or 344SQ_miR-200 primary tumours 6 weeks post subcutaneous injection of cancer cells into 129/Sv mice. Representative Ki67 or GzB staining in an individual tumour sample is shown on the left, and mean Ki67+or GzB+populations of gated CD8+T cells in total T cells are shown on the right (n=5). (e) CD8+T-cell depletion results in tumour growth and metastasis in mice (n=5) that received subcutaneous tumour cell injections. No treatment (344SQ_vector (Vector)), IgG (344SQ_miR-200+IgG control), or Ab (344SQ_miR-200+anti-CD8 Ab). The analysis was done 6 weeks post injection. (f) Relative abundance of CD8+T cells in the tumour (left) or lung (right) from 129/Sv mice (n=5) with syngeneic control 344SQ tumours (Vector), 344SQ_miR-200 tumours with control IgG treatment (IgG) or anti-CD8 antibody treatment (Ab). (g) Lung metastases of 344SQ_vector (Vector) and 344SQ_miR-200 (miR-200) tumours in WT or 129/SvRag2−/−(Rag2−/−) mice (n=5). The analysis was done 6 weeks post tumour cell subcutaneous injection. All the analyses were independently repeated twice. Data are shown as mean±s.e.m.t-test was used to analyze the data, withPvalues shown in the graphs. Figure 4: The miR-200/ZEB1 axis controls tumour metastasis through regulating CD8 + TILs. ( a , b ) Fluorescence-activated cell sorting analysis of ( a ) CD8 + TIL frequency, ( b ) PD1 and TIM3 marker expression on CD8 + T cells from 393P_vector and 393P_ZEB1 ( n =5), as well as 344SQ_vector and 344SQ_miR-200 ( n =10) primary tumours. Analysis was done 2 weeks post cancer cell injection. ( c , d ) Intratumoral Ki67 + CD8 + T cells ( c ); granzyme B (GzB) + CD8 + T cells ( d ) in 344SQ_vector or 344SQ_miR-200 primary tumours 6 weeks post subcutaneous injection of cancer cells into 129/Sv mice. Representative Ki67 or GzB staining in an individual tumour sample is shown on the left, and mean Ki67 + or GzB + populations of gated CD8 + T cells in total T cells are shown on the right ( n =5). ( e ) CD8 + T-cell depletion results in tumour growth and metastasis in mice ( n =5) that received subcutaneous tumour cell injections. No treatment (344SQ_vector (Vector)), IgG (344SQ_miR-200+IgG control), or Ab (344SQ_miR-200+anti-CD8 Ab). The analysis was done 6 weeks post injection. ( f ) Relative abundance of CD8 + T cells in the tumour (left) or lung (right) from 129/Sv mice ( n =5) with syngeneic control 344SQ tumours (Vector), 344SQ_miR-200 tumours with control IgG treatment (IgG) or anti-CD8 antibody treatment (Ab). ( g ) Lung metastases of 344SQ_vector (Vector) and 344SQ_miR-200 (miR-200) tumours in WT or 129/Sv Rag2 −/− ( Rag2 −/− ) mice ( n =5). The analysis was done 6 weeks post tumour cell subcutaneous injection. All the analyses were independently repeated twice. Data are shown as mean±s.e.m. t -test was used to analyze the data, with P values shown in the graphs. Full size image Because CD8 + T-cell infiltration affected not only metastasis but also the growth of primary tumours ( Fig. 4e and Table 1 ), we examined whether the effects of CD8 + T cells on metastasis depend on primary tumour size. Adjusted numbers of 344SQ, 344SQ_miR-200 and 393P tumour cells were injected into 129/SV mice to allow the primary subcutaneous tumours to grow to a similar size. The mice were killed 6 weeks post injection when the primary tumour masses reached 800–1,000 mg in size, and lung metastases were examined. Significant differences in lung metastasis were observed, even though the primary tumours were of similar size ( Supplementary Fig. 6a,b ). In a complementary experiment, we found that the number of CD8 + T cells and the percentage of PD1 + TIM3 + exhausted T cells were strictly dependent on metastatic potential, not on primary tumour size ( Supplementary Fig. 6c–e ). In addition, metastatic potentials of the different cell lines following injection with the same cell number via the tail vein were the same as with subcutaneous injection ( Supplementary Fig. 6f ), further indicating that metastatic potential was not dependent on the primary tumour mass. Furthermore, miR-200 levels in tumour cells did not affect the numbers of CD8 + T cells in the spleen and peripheral blood, nor did it affect CD8 + T-cell migration in vitro , suggesting that miR-200 controls the local abundance of CD8 + TILs in the tumour microenvironment without affecting CD8 + T-cell recruitment. Collectively, our data demonstrated that metastatic potential is dependent on the miR-200 levels in KP tumours, which determine the abundance and function of CD8 + TILs, independent of primary tumour size, growth rate or route of inoculation. miR-200/ZEB1 regulating CD8 + TIL function is PD-L1 dependent To determine whether cancer cell-autonomous PD-L1 directly induces CD8 + TIL exhaustion and tumour metastasis, we depleted PD-L1 in 344SQ cells by short hairpin RNA (shRNA)-mediated knockdown ( Fig. 5a ) and tested them in syngeneic mice. Primary tumour size and number of lung metastases in 344SQ-shPD-L1-bearing mice were significantly reduced relative to control transfectants ( Fig. 5b ), along with a fourfold increase in CD8 + T cells and a decrease in the percentage of exhausted CD8 + TILs (PD1 + TIM3 + and PD1 + LAG3 + ; Fig. 5c,d ). Similarly, PD-L1 neutralization in mice bearing implanted 344SQ and 393P_ZEB1 tumours by intraperitoneal injection of an anti-PD-L1 antibody reduced tumour size, metastasis and exhausted CD8 + T cells relative to control IgG ( Fig. 6a–c ), and increased infiltrating CD8 + T cells, intratumoral Ki67 + and granzyme B + CD8 + T cells ( Fig. 6d and Supplementary Fig. 7 ). On the other hand, the anti-PD-L1 antibody treatment did not show significant effects on tumours with constitutively high miR-200 levels (344SQ_miR-200 and 393P) ( Fig. 6 ). Consistent with these findings, when PD-L1 was genetically reconstituted into 344SQ_miR-200 and 344SQ-shPD-L1 cells, the primary subcutaneous tumours grew larger, had less CD8 + TILs and more exhausted T cells and produced more metastatic lungs nodules ( Supplementary Fig. 8 ). We thus conclude that miR-200 downregulation increases PD-L1 tumour cell expression, which drives CD8 + T-cell suppression in the tumour microenvironment and facilitates metastasis. 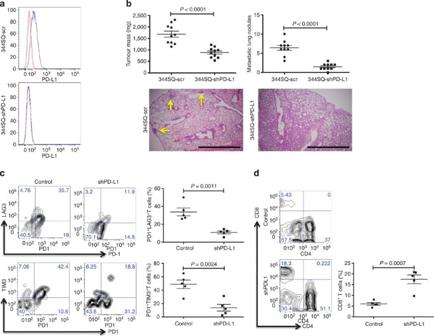Figure 5: Genetic targeting of PD-L1 expression on cancer cells reverses the CD8+TIL dysfunction and suppresses metastasis. (a) Cell surface expression of PD-L1 on 344SQ PD-L1 knockdown (344SQ-shPD-L1) versus 344SQ scramble control (344SQ-scr) cells by fluorescence-activated cell sorting (FACS; red line, isotype control staining; blue line, anti-PD-L1 staining). The measurement was independently repeated at least three times. (b) Primary tumour mass (top left) and lung metastases (top right) in 129/Sv mice (n=10) injected subcutaneously with 344SQ-shPD-L1 or 344SQ-scr cancer cells. Micrometastases (bottom) observed in haematoxylin and eosin-stained lung tissue sections are indicated by yellow arrows. Scale bar, 2 mm. Samples were obtained 6 weeks post injection. The data from two independent experiments were pooled. Data are shown as mean±s.e.m.t-test was used to analyze the data.Pvalues are shown in the graphs. (c,d) FACS analysis of (c) surface PD1, LAG3 and TIM3 marker expression levels on CD8+T cells; (d) CD8+TIL frequency for primary tumours in 129/Sv mice (n=5) injected subcutaneously with 344SQ-shPD-L1 (shPD-L1) or 344SQ-scr control (Control) cancer cells and necropsied 2 weeks later. The analyses were independently repeated three times. Data are shown as mean±s.e.m.t-test was used to analyze the data.Pvalues are shown in the graphs. Figure 5: Genetic targeting of PD-L1 expression on cancer cells reverses the CD8 + TIL dysfunction and suppresses metastasis. ( a ) Cell surface expression of PD-L1 on 344SQ PD-L1 knockdown (344SQ-shPD-L1) versus 344SQ scramble control (344SQ-scr) cells by fluorescence-activated cell sorting (FACS; red line, isotype control staining; blue line, anti-PD-L1 staining). The measurement was independently repeated at least three times. ( b ) Primary tumour mass (top left) and lung metastases (top right) in 129/Sv mice ( n =10) injected subcutaneously with 344SQ-shPD-L1 or 344SQ-scr cancer cells. Micrometastases (bottom) observed in haematoxylin and eosin-stained lung tissue sections are indicated by yellow arrows. Scale bar, 2 mm. Samples were obtained 6 weeks post injection. The data from two independent experiments were pooled. Data are shown as mean±s.e.m. t -test was used to analyze the data. P values are shown in the graphs. ( c , d ) FACS analysis of ( c ) surface PD1, LAG3 and TIM3 marker expression levels on CD8 + T cells; ( d ) CD8 + TIL frequency for primary tumours in 129/Sv mice ( n =5) injected subcutaneously with 344SQ-shPD-L1 (shPD-L1) or 344SQ-scr control (Control) cancer cells and necropsied 2 weeks later. The analyses were independently repeated three times. Data are shown as mean±s.e.m. t -test was used to analyze the data. P values are shown in the graphs. 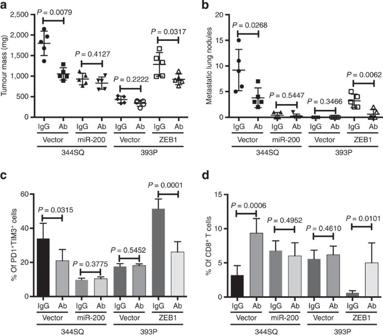Figure 6: Pharmacologic targeting of PD-L1 with antibody treatment prevents tumour growth and metastasis. (a,b) The tumour burden (a) and lung metastases (b) 6 weeks post cancer cell injection into 129/Sv mice (n=5) with IgG control (IgG) or anti-PD-L1 antibody (Ab) treatment. Anti-PD-L1 antibody or IgG control was injected (100 μg, intraperitoneally) twice a week for 6 weeks after the subcutaneous tumour cell injection. Following killing, mice were necropsied to harvest primary tumours and lungs, which were weighed, and to quantify distant metastases. (c,d) The CD8+T-cell function and the abundance of CD8+T cells in tumours (n=5) after anti-PD-L1 antibody treatment. All the analyses were independently repeated twice. Data are shown as mean±s.e.m.t-test was used to analyze the data.Pvalues are shown in the graphs. Full size image Figure 6: Pharmacologic targeting of PD-L1 with antibody treatment prevents tumour growth and metastasis. ( a , b ) The tumour burden ( a ) and lung metastases ( b ) 6 weeks post cancer cell injection into 129/Sv mice ( n =5) with IgG control (IgG) or anti-PD-L1 antibody (Ab) treatment. Anti-PD-L1 antibody or IgG control was injected (100 μg, intraperitoneally) twice a week for 6 weeks after the subcutaneous tumour cell injection. Following killing, mice were necropsied to harvest primary tumours and lungs, which were weighed, and to quantify distant metastases. ( c , d ) The CD8 + T-cell function and the abundance of CD8 + T cells in tumours ( n =5) after anti-PD-L1 antibody treatment. All the analyses were independently repeated twice. Data are shown as mean±s.e.m. t -test was used to analyze the data. P values are shown in the graphs. Full size image Intratumoral CD8 + T-cell activity is dynamically modulated through diverse mechanisms including loss of tumour cell antigenicity, changes in the expression of B7 family T cell co-inhibitory molecules (PD-L1 and PD-L2) and co-stimulatory molecules (CD80, CD86 and MHC class II) on tumour cells and the recruitment and activation of a variety of intratumoral immune cells [19] , [20] , [21] . Flow cytometric analysis of high- versus low-miR-200 tumours demonstrated no evidence of enhanced recruitment of myeloid-derived suppressor cells (CD11b + Gr-1 + ) or tumour-associated macrophages (CD11b + CD11c + Gr-1 + ). Constitutive miR-200 expression in 344SQ cells did not increase MHC class I expression or enhance CD8 + T cell-mediated tumour cell cytotoxicity in cell-killing assays, arguing against altered tumour cell antigenicity affecting CD8 + TIL-mediated tumour rejection. On the basis of the extensive studies of IFN-γ, it is well known that this cytokine plays a key role in tumour surveillance [29] and is a potent inducer of PD-L1 expression, which was proposed as a cause of tumour immune evasion [25] . We questioned whether the miR-200/ZEB1 axis modulates the IFN-γ pathway through the regulation of Janus Kinase/Signal Transducer and Activator of Transcription signalling, but found no signalling pathway changes to support this ( Supplementary Fig. 9a ). We then tested the impact of IFN-γ blockade on tumour growth in vivo . On treatment with a neutralizing IFN-γ antibody, PD-L1 expression on mesenchymal (344SQ) tumours dramatically decreased ( Supplementary Fig. 9b ), while both the mesenchymal (344SQ) and epithelial (344SQ_miR-200) syngeneic tumours showed increased growth, with a dramatic decrease in total CD8 + TILs ( Supplementary Fig. 9c,d ). However, within the IFN-γ-blocking antibody group, there was still a significant difference between miR-200 high and miR-200 low tumours in growth, CD8 + TILs and exhausted T cells ( Supplementary Fig. 9c–e ). In addition, with IFN-γ blockade, there was a significant decrease in exhausted T cells in mesenchymal tumours, while there was no significant decrease in epithelial tumours ( Supplementary Fig. 9e ), again emphasizing that mesenchymal tumours are more sensitive to IFN-γ. Taken overall, the data demonstrates that the miR-200/ZEB1 axis is a downstream regulator of PD-L1 that can modulate the effects of the IFN-γ pathway. Repression of antitumour immunity requires tumour cell PD-L1 Diverse cell types in the tumour microenvironment (for example, myeloid cells, fibroblasts and endothelial cells) express PD-L1, which could suppress antitumour immunity in the absence of tumour cell PD-L1 expression. However, when multiple different cancer cell types (B16 melanoma, KPC pancreas or MC38 colon) were implanted into PD-L1 WT and knockout (KO) mice, there was no significant difference in tumour growth between WT and KO mice ( Supplementary Fig. 10 ). To determine whether the expression on other cell types rescues PD-L1 deficiency on tumour cells, we utilized the Lewis lung carcinoma (LLC) model in which, based on the treatment with anti-PD-L1 antibody, PD-L1 promotes primary tumour growth and metastasis ( Supplementary Fig. 11 ). In addition, miR-200 represses PD-L1 expression in the LLC model as in the KP model ( Supplementary Fig. 12a ). We generated LLC cell lines with intermediate or very low level PD-L1 expression using shRNA to PD-L1 ( Fig. 7a ), injected these cells into WT or PD-L1-KO mice ( Fig. 7b ) and measured tumour growth rate ( Fig. 7c ), intratumoral CD8 + T cells ( Fig. 7d ), mouse survival, final tumour weight and number of metastases ( Supplementary Fig. 12b–d ). PD-L1 deficiency in tumour cells suppressed tumour growth and metastasis and increased intratumoral CD8 + T cells, which were reversed by stable reconstitution of PD-L1 in the shPDL1 LLC cells ( Fig. 7e,f ). In contrast, PD-L1 deficiency in the host had no detectable effect on PD-L1-deficient or -replete LLC tumours ( Fig. 7a–f and Supplementary Fig. 12b–d ). We conclude that PD-L1 expression on tumour cells plays a dominant role in the regulation of CD8 + T cell-mediated antitumour immunity. 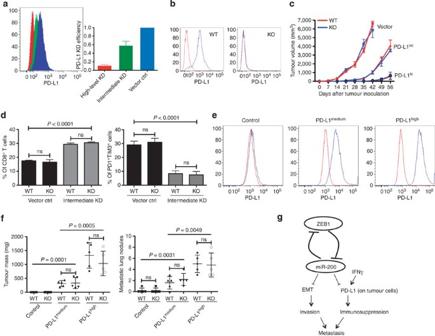Figure 7: PD-L1 expression on tumour cells is critical to the repression of antitumour immunity. (a) The knockdown (KD) efficiency of PD-L1 in LLC-JSP murine lung cancer cells measured by fluorescence-activated cell sorting (FACS). Representative histograms (left), and statistical analysis (right). The measurement was independently repeated at least three times. (b) Representative FACS histogram of PD-L1 expression on myeloid cells (CD11b+) in PD-L1-KO or WT mice (n=3). (c) Tumour growth in PD-L1-KO or WT mice (n=6) of subcutaneously injected LLC-JSP cells (10, 000 cells with 100 μl of PBS per mouse) with differing PD-L1 knockdown (Vector, PD-L1 KD vector control; PD-L1int, PD-L1 intermediate KD; PD-L1hi, PD-L1 high level KD). The data are shown from two independent experiments. Data are shown as mean±s.e.m. (d) FACS analysis of CD8+TIL frequency and T-cell exhaustion marker expression levels on CD8+T cells in subcutaneous primary tumours of LLC-JSP vector control (Vector ctrl) and LLC-JSP intermediate PD-L1 knockdown (Intermediate KD) in PD-L1 WT (WT) and PD-L1-KO (KO) mice (n=5, from two independent experiments). Analysis was done 3 weeks post tumour cell injection (20,000 cells with 100 μl of PBS per mouse).t-test was used to analyze the data.P<0.0001. (e) PD-L1 expression levels on LLC-JSP-shPD-L1 cells (the high knockdown efficiency cells) after reconstitution of PD-L1. The measurement was independently repeated at least three times. Control, LLC-JSP-shPD-L1+vector control; PD-L1medium, LLC-JSP-shPD-L1+intermediate overexpression of PD-L1; PD-L1high, LLC-JSP-shPD-L1+high overexpression of PD-L1. (f) Primary tumour masses and lung metastases in PD-L1-KO or WT mice (n=5) injected subcutaneously with the different reconstituted cell lines. Analysis was done 4 weeks post subcutaneous cancer cell injection (10,000 cells with 100 μl of PBS per mouse). The analyses were independently repeated twice. Data are shown as mean±s.e.m.t-test was used to analyze the data. NS,P>0.05. (g) The working model of the mutual regulation of EMT and immune suppression by miR-200/ZEB1 axis and their complementary role in metastasis. Figure 7: PD-L1 expression on tumour cells is critical to the repression of antitumour immunity. ( a ) The knockdown (KD) efficiency of PD-L1 in LLC-JSP murine lung cancer cells measured by fluorescence-activated cell sorting (FACS). Representative histograms (left), and statistical analysis (right). The measurement was independently repeated at least three times. ( b ) Representative FACS histogram of PD-L1 expression on myeloid cells (CD11b + ) in PD-L1-KO or WT mice ( n =3). ( c ) Tumour growth in PD-L1-KO or WT mice ( n =6) of subcutaneously injected LLC-JSP cells (10, 000 cells with 100 μl of PBS per mouse) with differing PD-L1 knockdown (Vector, PD-L1 KD vector control; PD-L1 int , PD-L1 intermediate KD; PD-L1 hi , PD-L1 high level KD). The data are shown from two independent experiments. Data are shown as mean±s.e.m. ( d ) FACS analysis of CD8 + TIL frequency and T-cell exhaustion marker expression levels on CD8 + T cells in subcutaneous primary tumours of LLC-JSP vector control (Vector ctrl) and LLC-JSP intermediate PD-L1 knockdown (Intermediate KD) in PD-L1 WT (WT) and PD-L1-KO (KO) mice ( n =5, from two independent experiments). Analysis was done 3 weeks post tumour cell injection (20,000 cells with 100 μl of PBS per mouse). t -test was used to analyze the data. P <0.0001. ( e ) PD-L1 expression levels on LLC-JSP-shPD-L1 cells (the high knockdown efficiency cells) after reconstitution of PD-L1. The measurement was independently repeated at least three times. Control, LLC-JSP-shPD-L1+vector control; PD-L1 medium , LLC-JSP-shPD-L1+intermediate overexpression of PD-L1; PD-L1 high , LLC-JSP-shPD-L1+high overexpression of PD-L1. ( f ) Primary tumour masses and lung metastases in PD-L1-KO or WT mice ( n =5) injected subcutaneously with the different reconstituted cell lines. Analysis was done 4 weeks post subcutaneous cancer cell injection (10,000 cells with 100 μl of PBS per mouse). The analyses were independently repeated twice. Data are shown as mean±s.e.m. t -test was used to analyze the data. NS, P >0.05. ( g ) The working model of the mutual regulation of EMT and immune suppression by miR-200/ZEB1 axis and their complementary role in metastasis. Full size image During the initial stages of metastasis, epithelial tumour cells undergo EMT, causing a loss of cell–cell contacts, increased motility and invasion into the surrounding stroma [33] . Occurring in parallel are changes in the tumour microenvironment that suppress antitumour immunity [11] . Although the synchronicity of these distinct biological processes implies the possibility of a common genetic driver, the existence of a molecular linkage between them has not been reported. Here we provide evidence that EMT is tied to the suppression of antitumour immunity through miR-200/ZEB1, an EMT regulatory axis that controls PD-L1 expression on tumour cells. Due to the double-negative feedback loop between ZEB1 and miR-200 that governs a reversible switch between epithelial and mesenchymal states [7] , [9] , [10] , we previously investigated the role of the miR-200/ZEB1 axis in the metastasis of lung adenocarcinoma and found that the ZEB1-induced suppression of miR-200 promotes tumour cell invasion and metastasis [2] , [28] , [32] . Since its discovery as a master regulator of EMT, the miR-200 family was subsequently found to regulate a number of complementary cellular functions relevant to tumour growth and metastasis, including stem cell properties, sensitivity to chemotherapeutic agents, reduction in angiogenesis and responsiveness to proapoptotic signals. The target genes identified to date through which miR-200 regulates these biologic properties are in most cases non-overlapping [34] , [35] , [36] , [37] , [38] , [39] , [40] , [41] . Similarly, studies on miR-31 have demonstrated that multitasking is an essential feature of its capacity to promote metastasis; concurrent re-expression of three target genes ( ITGA5 , RDX and RHOA ) is required to abrogate miR-31-imposed metastasis suppression [42] . Among its pleiotropic targets controlling complementary tumour cell functions, here we demonstrate that PD-L1 is a downstream target of the miR-200/ZEB1 axis and contributes to immunosuppression in the primary tumour tissue. Although the miR-200/ZEB1 axis regulation of PD-L1 may not entirely account for the immunosuppressive effects observed, PD-L1 blockade significantly improves CD8 + T-cell infiltration, reverses the exhausted T-cell phenotype, reduces tumour burden and metastases only with mesenchymal tumours (344SQ, 531LN2, 393P_ZEB1 and LLC-JSP) and not with epithelial tumours (344SQ_miR-200 and 393P; Figs 6 , 7 and Supplementary Figs 7, 11 and 12c,d ), while the reconstitution of PD-L1 expression reverses the phenotype of epithelial tumours (344SQ_miR-200, 344SQ-shPD-L1 and LLC-JSP-shPD-L1) ( Fig. 7e,f and Supplementary Fig. 8 ). We additionally observed that even in the absence of IFN-γ mesenchymal tumours produce T-cell exhaustion due to miR-200/ZEB1-regulated change of PD-L1 expression ( Supplementary Fig. 9b–e ), indicating that mesenchymal tumour cells are hardwired to prevent immune attack. However, there was a synergy between IFN-γ stimulation and miR-200 repression, illustrating how different modes of PD-L1 regulation can converge in the same tumour cells. These findings represent a remarkable departure from the tumour cell-autonomous processes regulated by the pleiotropic miR-200 family and are, to our knowledge, the first example of a microRNA expressed in tumour cells that regulates metastasis by modulating intratumoral immune cell function. The convergence of these biological processes on a single microRNA presents a clear selective advantage to tumour cells in which this microRNA is silenced, as shown in the model ( Fig. 7g ). The dynamic interaction of immune and cancer cells in tumour tissues plays a critical role in controlling cancer progression. Among the various immune cell infiltrates into tumour tissues, CD8 + TILs appear to be the key immune cells showing strong cytotoxic activity that is direct and selective for cancer cells [43] . Survival duration correlates positively with intratumoral CD8 + T-cell abundance and negatively with intratumoral expression of the T-cell co-inhibitory molecule PD-L1 and its receptor PD1, providing strong clinical relevance of prognostic value in patients with various epithelial tumour types, including lung cancer [44] , [45] , [46] . Furthermore, PD-L1/PD1 axis blockade in preclinical models, including those reported here, suppresses tumour growth and metastasis [44] , [45] . However, PD-L1 is expressed on multiple intratumoral cell types that may cooperate to effect CD8 + T-cell suppression. Here we addressed the relative importance of different cellular sources of PD-L1 to assess whether PD-L1 upregulation on tumour cells alone is sufficient to cause CD8 + T-cell immunosuppression ( Fig. 7 and Supplementary Figs 8 and 12b–d ). We found that intratumoral CD8 + T-cell exhaustion is mediated primarily by tumour cell PD-L1 expression. PD-L1 on tumour cells, rather than other cell types, results in CD8 + T-cell exhaustion and diminution of CD8 + TIL number in a chronic fashion. The finding that other cell types exerted no measurable effect was surprising but may not be unique to the models studied in depth here as multiple different tumour models show a similar effect ( Figs 5 and 7 and Supplementary Figs 8 and 12 ), which serves to illustrate the point that miR-200/ZEB1 controls metastasis in part through tumour cell non-autonomous mediators. Patients with advanced melanoma experience a survival advantage following CD8 + T-cell reactivation by treatment with antibodies targeting CTLA-4, another B7-CD28 family member [47] . Evidence from lung cancer preclinical models presented here and elsewhere [48] that PD-L1-induced CD8 + T-cell exhaustion promotes tumour growth and metastasis raises the possibility that treatment with PD-L1 inhibitors might provide therapeutic benefit to lung cancer patients. Clinical trials with anti-PD-L1 or PD1-neutralizing antibodies are ongoing in patients with a variety of solid tumours, including lung cancer, with preliminary data indicating significant benefit for subsets of lung cancer patients with established metastatic disease [49] . Such strategies might be combined with anti-CD25 antibodies that deplete CD4 + Foxp3 + regulatory T cells, which enhance the antitumour efficacy of cytotoxic chemotherapy in lung cancer preclinical models [50] . On the basis of evidence presented here that PD-L1 is upregulated in early-stage lung adenocarcinomas that have a mesenchymal expression pattern and low miR-200 expression, representing up to one-third of patients, it is tempting to speculate that PD-L1 inhibitors will be particularly efficacious in this group of patients. Human samples The initial set of samples analysed consisted of lung adenocarcinoma cases from The Cancer Genome Atlas (TCGA) project ( http://cancergenome.nih.gov/ ) [27] , which represent early-stage surgical resection specimens and were collected in accordance with The Cancer Genome Atlas (TCGA) Human Subjects Protection and Data Access Policies. The second set of samples was from the Department of Thoracic/Head and Neck Medical Oncology at MD Anderson. The Profiling of Resistance patterns and Oncogenic Signaling Pathways in Evaluation of Cancers of the Thorax (PROSPECT) trial was developed in 2006 with the purpose of investigating molecular mechanisms of therapeutic resistance, and was recently completed. After MDACC Institutional Review Board approval of the protocol, retrospectively identified samples were collected from two hundred and fifteen patients enrolled in the PROSPECT trial. Stage distribution varied, but almost all patients had locoregionally confined disease, as expected from a set of specimens from surgical resection. For each dataset, an EMT score for each sample was computed using an averaging scheme based on mRNA expression of 76 EMT signature genes previously published by our group [26] . The scores were calculated as the average expression level of mesenchymal genes minus the average expression level of epithelial genes. Plasmids and reagents pLenti4.1-miR-200 was obtained from Dr Gregory Goodall (University of Adelaide) and used as described elsewhere [2] , [7] , [28] . A modified doxycycline-inducible pTRIPz-RFP vector expressing miR-200a, miR-200b or in combination (miR-200ab) was generously provided to us by Dr Gregory Goodall at the University of Adelaide. Mouse ZEB1 was subcloned into pcDNA3.1/His C (Invitrogen) to generate the ZEB1 overexpression vector. shRNA to mouse ZEB1 and PD-L1 and scrambled controls in the pGFP-V-RS vector were obtained from OriGene. Mouse PD-L1 expression vector pUNO1-mCD274 was purchased from Invivogen. Pre-microRNAs miR-200c and negative control (scrambled oligos) (Life Technologies) were reverse transfected into cells with Lipofectamine 2000 (Life Technologies) at a final concentration of 50 nM. siRNA knockdown for PD-L1 expression analysis Cells seeded in a six-well plate were transfected with siRNA of ZEB1 (40 nM; OriGene) as well as their scrambled controls. The cells were collected 48 h after transfection to examine PD-L1 expression. PD-L1 3′-UTR reporter assay miRNA-binding sites were predicted by TargetScan (release 5.1; http://www.targetscan.org ). Human CD274 (4.6 kb) was cloned by PCR and ligated into the pCI-neo-hRL vector. The ZEB1 3′-UTR (1.9 kb) subcloned into the same vector was used as a control. Mutation of the individual miR-200 sites (Mut A or Mut B) or a double mutant at both sites was made and cloned into the same vector. These reporters were cotransfected with individual synthetic miR-200 family precursors (5 nM; Ambion) into either murine 344SQ, or human H1299 or H157 cells (1.0 × 10 5 cells per well) in 24 well plates. pGL3-basic (50 ng; Promega) was used as an internal control. Forty-eight hours post transfection, dual-luciferase activity was measured with the Dual-Luciferase Reporter Assay System (Promega). Results were normalized on the basis of firefly luciferase according to the manufacturer’s protocol. Cells and mice The epithelial 393P and 393LN as well as mesenchymal 344P, 344SQ, 531LN2 and 531LN3 cell lines were derived from KP mice [27] , [51] . B16 melanoma, KPC pancreatic and MC38 colon, LLC-JSP Lewis lung cancer cell lines were maintained in our laboratories. Stable cell lines 344SQ_miR-200, 531LN2_miR-200 and H1155_miR-200 were generated by pLenti4.1-miR-200 lentivirus transduction. H157 cells were transduced by lentiviral delivery of the doxycycline-inducible pTRIPz-miR-200 or control vector (miR-200a, b or ab). Stable cell lines 344SQ-shPD-L1 and LLC-JSP-shPD-L1 were generated by transfection with shRNA expression vectors. Stable cell lines 393P_ZEB1 and HCC827_ZEB1 were generated by transfection with the corresponding expression vectors. Stable cell lines PD-L1-expressing 344SQ_miR-200, PD-L1-overexpressed 344SQ-shPD-L1 and PD-L1-overexpressed LLC-JSP-shPD-L1 were generated with mouse PD-L1 expression vector pUNO1-mCD274 (Invivogen). Stable cell line LLC-JSP-t2 was generated in our laboratory. Human lung cancer H322, H1299, H441, H157, H1155, HCC827 and H460 cell lines were purchased from the American Type Culture Collection. The H460 and H1299 cells with stable shRNA-mediated knockdown of ZEB1 were kindly provided by Dr Raymond E. Meyn (Professor, Department of Experimental Radiation Oncology, Division of Radiation Oncology, The University of Texas MD Anderson Cancer Center, Houston, TX). Six- to 8-week-old 129/Sv or C57BL/6 male mice were obtained from Charles River Laboratories; 129/Sv Rag2 −/− mice were obtained from Taconic and 6- or 8-week-old male mice were used for the experiments. PD-L1-deficient C57/BL6 mice were obtained from L. Chen lab and maintained as a homozygous line and 6- or 8-week-old male mice were used for the experiments. Spontaneous K-ras and K-ras/p53 mice were generated by our laboratory [52] . Eight- to 12- month-old K-ras and K-ras/p53 mice were used for the experiments. All animal procedures were reviewed and approved by the University of Texas MD Anderson Cancer Center Animal Care and Use Committee. Tumour models For examining intratumoral lymphocyte populations, 2 × 10 6 cancer cells in 100 μl of 50% Growth Factor Reduced BD Matrigel Matrix (BD Biosciences) were subcutaneously injected into the flanks of 129/Sv mice. If not specified otherwise, tumours were harvested and analysed 2 weeks after injection. For studying the growth rate of the primary tumour mass and formation of lung metastases, if not indicated, 1 × 10 6 cancer cells in 100 μl of PBS were injected subcutaneously into the mouse flank. For the orthotopic model, 1 × 10 6 cancer cells were mixed with a 1:10 dilution of Matrigel and injected into the lung as described elsewhere [53] . Mice were monitored regularly and killed 5–6 weeks after the tumour cell injections. At end points, mice were killed to examine the primary and metastatic tumours. For studying the relationship of the primary subcutaneous tumour and the lung metastasis, 1 × 10 6 344SQ cells, 2 × 10 6 344SQ_miR-200 cells or 3 × 10 6 393P cells in 100 μl of PBS were injected subcutaneously into 129/Sv mice. Mice with comparable sizes of primary tumours were chosen for examining lung metastasis at necropsy 6 weeks after injection. For experimental pulmonary metastasis, 5 × 10 5 cancer cells were injected through the tail vein. Lungs were removed to measure metastatic nodules 6 weeks later. For lung metastasis measurement, except for LLC-JSP-t2-bearing lungs, in which the metastatic lung nodules were counted under the fluorescent microscope, the lungs were removed and immersed in cold PBS for 2–3 h, the grey nodules on the surface of lung were counted as described previously [52] , [53] . Antibody-mediated cell depletion Anti-CD8 antibody (2.43; BioXCell) or an immunoglobulin G (IgG) control was injected into the mice (200 μg, intraperitoneally) twice weekly for 2 weeks beginning on day 1 after a subcutaneous cancer cell injection. CD8 T cell adoptive transfer CD8 + T cells were isolated from splenocytes of 129/Sv mice by MACS technology according to the manufacturer’s instructions (Miltenyi Biotec). CD8 + T cells (4 × 10 6 ) were injected via the tail vein into 129/Sv Rag2 −/− mice 48 h before tumour inoculation. Anti-PD-L1 and anti-IFN-γ antibody neutralization Anti-PD-L1 (9G2; BioXcell) antibody or an isotype-matched IgG control was injected into 129/Sv or C57BL/6 mice (100 μg, intraperitoneally) twice a week for 3 or 6 weeks beginning on day 1 after the subcutaneous indicated tumour cell injection. 129/Sv mice were treated on days −1, +2 and +5 with intraperitoneal injections of 250 μg of neutralizing antibody to murine IFN-γ (XMG1.2; BioXcell) as described [29] . Flow cytometry Single-cell suspensions were prepared and stained according to standard protocols for flow cytometry with the following antibodies: mouse CD3-PerCP (BD Biosciences, 560527 1:100 dilution), CD4-APC (mouse; BD Biosciences, 553051, 1:100 dilution), CD4-FITC (mouse; BD Biosciences, 553729, 1:50 dilution), CD8b-APC (mouse; eBioscience, 17-0083, 1:100 dilution), CD8b-PE (mouse; eBioscience, 12-0083-83, 1:200 dilution), CD11b-APC (mouse; eBioscience, 17-0112-83, 1:100 dilution), Ki67-PE (eBioscience, 12-5698-82, 1:100 dilution), GzB-PE (eBioscience, 12-8898-82, 1:100 dilution), PD1-PE (mouse; eBioscience, 12-9985-83, 1:150 dilution), PD1-FITC (mouse; eBioscience, 11-9985-82, 1:150 dilution), PD-L1-PE (mouse; BD Biosciences, 558091, 1:200 dilution), PD-L1-PE (human; eBioscience, 12-5983-42, 1:200 dilution), TIM3-PE (mouse; eBioscience, 12-5870-83, 1:150 dilution), and LAG3-PE (mouse; eBioscience, 12-2231-83, 1:100 dilution). For intracellular staining, cells were fixed and permeabilized with BD Cytofix/Cytoperm (BD Biosciences). The data were acquired on a Fortessa or Calibur platform (BD Biosciences) and analysed with FlowJo software (version 7.6; Tree Star). For analysing the abundance and the function of CD4 + or CD8 + TILs, single-cell suspensions were prepared from tumours and inguinal lymph nodes and stained; the staining of inguinal lymph node cells was used as the reference of lymphocyte gating, then CD3 + cells were gated, and then CD4 + or CD8 + population was analysed. RNA and protein analyses Total RNA was isolated from cultured cells with TRIzol (Invitrogen). cDNA was synthesized by using the SuperScript III kit (Invitrogen), and qPCR was done with the SYBR Green PCR Master Mix (Applied Biosystems). Primers were designed with National Center for Biotechnology Information (NCBI) primer design software. Relative expression levels were normalized by B2M and calculated by the 2 −ΔΔ C t method [54] . The primers used for qPCR are shown in Supplementary Table 3 (mZEB1, hZEB1, mPD-L1, hPD-L1, hNcad, hEcad, hVim). miR-200 expression assays were performed using 10 ng of total RNA according to the manufacturer’s instructions (Applied Biosystems). Values were normalized on the basis of control miR-16 levels. Total protein was extracted using NP40 lysis buffer (0.5% NP40, 250 mM NaCl, 50 mM Hepes, 5 mM ethylenediaminetetraacetic acid, 0.5 mM egtazic acid) supplemented with protease inhibitors cocktails (Sigma-Aldrich). Lysates was centrifuged at 12,000 r.p.m. for 10 min, and the supernatant was collected for experiments. Protein lysates (40 μg) were resolved on denaturing gels with 4 to 20% SDS-polyacrylamide and transferred to nitrocellulose membranes (Biorad Laboratories). Membranes were probed with the following antibodies: primary antibodies anti-ZEB1 (Santa Cruz, sc-25388, 1:500 dilution), anti-Ncad (BD Biosciencses, 610921, 1:500 dilution), anti-Ecad (BD Biosciences, 610182, 1:10,000 dilution), anti-Vim (Cell Signaling, 3,932 s, 1:500 dilution), anti-STAT1 (Abcam, ab2415, 1:2,000 dilution), anti-p-STAT1 (Tyr 701) (Santa Cruz, sc-7988, 1:1,000 dilution), anti-p-STAT1 (Ser 727) (Abcam, ab109461, 1:1,000 dilution), anti-Jak1 (Abcam, ab75744, 1:1,000 dilution), anti-p-Jak1 (Tyr 1022/1023) (Santa Cruz, sc-16773, 1:1,000 dilution), anti-IFNGR1 (Santa Cruz, sc-702, 1:3,000 dilution), anti-Actin (Abcam, ab8227, 1:5,000 dilution) and secondary antibody labelled by horseradish peroxidase (Amersham GE Healthcare). The secondary antibody was visualized using a chemiluminescent reagent Pierce ECL kit (Thermo Scientific). The original photos of western blots are shown in Supplementary Fig. 13 . Histologic analysis Tissues were fixed in 10% paraformaldehyde and embedded in paraffin. Haematoxylin and eosin-stained sections were examined to identify micrometastases. For immunohistochemical, cryosections (8 μm) of tumour tissues were fixed with acetone and stained with antibody against mouse PD-L1 (Abcam, ab58810, dilution 1:100) and horseradish peroxidase-conjugated secondary antibody. Images (× 20) were acquired with an Olympus BX41 microscope. Statistics All statistical analyses were performed with GraphPad Prism 5.0 software. Significant differences ( P <0.05) between two groups were identified by Student’s t -tests. How to cite this article : Chen L., et al . Metastasis is regulated via microRNA-200/ZEB1 axis control of tumour cell PD-L1 expression and intratumoral immunosuppression. Nat. Commun. 5:5241 doi: 10.1038/ncomms6241 (2014).